Tactile stimulation lowers stress in fish In humans, physical stimulation, such as massage therapy, reduces stress and has demonstrable health benefits. Grooming in primates may have similar effects but it remains unclear whether the positive effects are due to physical contact or to its social value. Here we show that physical stimulation reduces stress in a coral reef fish, the surgeonfish Ctenochaetus striatus . These fish regularly visit cleaner wrasses Labroides dimidiatus to have ectoparasites removed. The cleanerfish influences client decisions by physically touching the surgeonfish with its pectoral and pelvic fins, a behaviour known as tactile stimulation. We simulated this behaviour by exposing surgeonfish to mechanically moving cleanerfish models. Surgeonfish had significantly lower levels of cortisol when stimulated by moving models compared with controls with access to stationary models. Our results show that physical contact alone, without a social aspect, is enough to produce fitness-enhancing benefits, a situation so far only demonstrated in humans. In humans and other vertebrates alike, positive social interactions in which physical contact is involved seem to be a primary coping strategy to decrease stress. Stress relief occurs by a reduction of the activity of the hypothalamic–pituitary–adrenal axis, which can be demonstrated by lowered circulating glucocorticoid levels (cortisol or corticosterone) [1] , [2] . Current opinion holds that a relatively quick increment in glucocorticoid levels from a low baseline in response to a stressor, followed by a fast induction of negative feedback, is a good indicator of a successful coping strategy and health status [3] . Otherwise, unpredictable and/or harmful situations may have long-lasting effects on an animal's endocrinological and metabolic states, which may consequently become detrimental to health [4] . A large body of work demonstrates that massage yields positive effects on health-related factors in humans, which translate in a reduction in stress as measured by cortisol levels [5] , [6] , [7] , [8] . These effects are largely due to physical contact, as massages in these studies were typically delivered by a stranger rather than by a socially close individual. In non-human primates, grooming seems to have similar positive effects, including the lowering of stress-related behavioural indices and the reduction of heart rate levels and neuroendocrine responses to stress [9] , [10] , [11] , [12] , [13] . However, it remains unclear whether in such taxa, the effects are due to physical contact alone or to the stabilizing effects of grooming on social relationships [9] , [14] , [15] . In favour of the latter hypothesis is the fact that stress reduction in primates has been linked to both receiving and providing grooming [11] , [13] . More–over, in wild female baboons, providing grooming seems to relieve stress responses during challenging situations, such as social instability [16] . Also in other mammals, the effects of touching versus relationship improvement cannot be easily separated. For instance, the physical stimulation of suckling and physical contact with their pups produces stress-reducing effects in female rats [17] , [18] . The discovery of a positive effect of physical contact in a reef fish, in addition to providing the first experimental evidence of its health benefits in a non-human, would resolve a long-standing paradox described in cleaning mutualism involving cleanerfish of the genus Labroides and their reef fish 'clients'. Clients frequently visit cleaners at specific sites or territories, known as cleaning stations, and signal that they wish to be inspected by posing (that is, adopting a species-specific immobile posture with all fins spread) [19] , [20] . Cleaners may cooperate by removing ectoparasites but they may also cheat by eating client mucus, which they prefer [21] , [22] but which is costly for clients to replace [22] . As a consequence, conflicts between cleaners and clients arise regularly [23] . In such situations, cleaners often straddle the back of their clients and provide a massage with their pelvic and pectoral fins—a behaviour termed tactile stimulation [24] . Cleaners use tactile stimulation in a variety of contexts, including to build relationships with new clients, to reconcile after having cheated and as a pre-conflict management strategy with predators [24] , [25] . Tactile stimulation seems to manipulate client behaviour as it increases the likelihood that clients will remain at a cleaning station and the time they spend interacting with cleaners [24] , [25] . The classic view has been that cleaners exploit the properties of the clients' sensory system and that clients gain little from tactile stimulation [26] . However, given the frequent occurrence of this behaviour and the potential costs to clients, it seems surprizing that selection would not have countered the cleaners' manipulation tactics. An alternative hypothesis is that clients accept tactile stimulation because it provides them with direct benefits. Here, we investigated how physical contact affects cortisol levels in a coral reef surgeonfish, the lined bristletooth C. striatus . Based on research demonstrating health benefits of physical contact in humans [5] , [6] , [7] , [8] , we assumed that similar benefits to clients should also be measurable at the physiological level. As interactions with cleaners affect the stress axis and immune activity of clients [27] , [28] , we asked whether physical contact alone, without the additional benefit of parasite removal, could contribute to a change in client stress levels, namely causing cortisol levels to decline. Twice a day, for a period of 10 days, we provided to captive surgeonfish, which are frequent visitors to cleaning stations in the wild [22] , access to a model cleanerfish, which had a soft brush on its ventral side. Models were either connected to a mechanized string, which enabled them to move back and forth (treatment), or they remained stationary (controls). Surgeonfish could then position themselves below the moving model and receive physical stimulation or not interact with the model ( Fig. 1 ). Fish behaviour with the models was recorded on the tenth day. We aimed to: investigate the influence of access to physical stimulation on surgeonfish captivity baseline cortisol levels; measure surgeonfish cortisol response to an unpredictable acute stress challenge (that is, exposure to confinement test). Half of the surgeonfish were exposed to moving models, the other half to stationary models, while half of each group was exposed to an acute stress challenge. We additionally evaluated whether cortisol levels correlated with the time surgeonfish spent interacting with the moving model. Our results have finally identified the elusive benefit to fish of receiving tactile stimulation from cleaners. We show that physical contact alone is enough to produce short-term benefits to client fish (reduction of stress levels). Moreover, our results suggest that pathways for sensory information processing should be rather uniform among vertebrates. 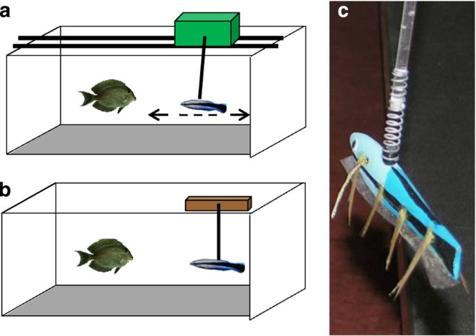Figure 1: Experimental set-up to test for the effect of physical stimulation on cortisol levels of surgeonfishC. striatus. (a) Individual fish exposed to a mechanical moving model of a cleaner fishL. dimidiatus(treatment); (b) Fish exposed to a stationary model (control), (c) A close-up of the cleaner wrasse model. On ten consecutive days, each fish was exposed to one of the two types of models for 2 h per day (1 h in the morning and 1 h in the afternoon). Figure 1: Experimental set-up to test for the effect of physical stimulation on cortisol levels of surgeonfish C. striatus . ( a ) Individual fish exposed to a mechanical moving model of a cleaner fish L. dimidiatus (treatment); ( b ) Fish exposed to a stationary model (control), ( c ) A close-up of the cleaner wrasse model. On ten consecutive days, each fish was exposed to one of the two types of models for 2 h per day (1 h in the morning and 1 h in the afternoon). Full size image Fish behaviour Surgeonfish readily approached the cleanerfish models ( Supplementary Movie 1 ). Surgeonfish with access to moving cleaner models posed (independent t test ( T i ), T i =2.57, df=25, P =0.02, Fig. 2a ), touched the model (single-contact events with model; T i =3.23, df=25, P =0.003, Fig. 2c ) and interacted with the model (engaged in continuous physical contact with the model: T i =3.45, df=25, P =0.005, Fig. 2b ) significantly more frequently than surgeonfish with access to stationary cleaner models. Similarly, surgeonfish spent a greater duration of time posing ( T i =2.48, df=25, P =0.03, Fig. 2d ) and interacting with moving models than with stationary ones ( T i =2.65, df=25, P =0.02, Fig. 2e ). 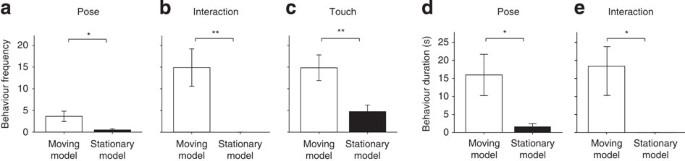Figure 2: Various behaviours of surgeonfishC. striatustowards cleanerfishL. dimidiatusmodels. Behaviour of surgeonfish with access to mechanically moving cleaner fish models (white bars,n=12 surgeonfish) and with access to stationary models (black bars,n=15). (a) Total number of fish-posing events (immobile posture with all fins spread with no contact with model), (b) total number of interaction events (longer touching events during which fish rubbed and was in continuous physical stimulation with the models), (c) total number of single-contact events with model (touch), (d) total duration of fish-posing events and (e) total duration of interaction events. Values were summed between the last two exposure sessions (1 h each) for each individual and then averaged across surgeonfish.P-values refer to independentt-tests (independentt-tests, *< 0.05; **< 0.01). Error bars represent±1 s.e.m. Figure 2: Various behaviours of surgeonfish C. striatus towards cleanerfish L. dimidiatus models. Behaviour of surgeonfish with access to mechanically moving cleaner fish models (white bars, n =12 surgeonfish) and with access to stationary models (black bars, n =15). ( a ) Total number of fish-posing events (immobile posture with all fins spread with no contact with model), ( b ) total number of interaction events (longer touching events during which fish rubbed and was in continuous physical stimulation with the models), ( c ) total number of single-contact events with model (touch), ( d ) total duration of fish-posing events and ( e ) total duration of interaction events. Values were summed between the last two exposure sessions (1 h each) for each individual and then averaged across surgeonfish. P -values refer to independent t -tests (independent t -tests, *< 0.05; **< 0.01). Error bars represent±1 s.e.m. Full size image Fish cortisol levels Surgeonfish that had access to physical stimulation, in the form of access to moving cleaner models, had lower cortisol plasma levels than those that had access to stationary cleaner models, regardless of confinement treatment (two-way analysis of variance (ANOVA) F 1,23 =4.65, P =0.04; Fig. 3 ). Confinement induced a stress response, with cortisol plasma levels being higher in the confined surgeonfish than in the unconfined fish, regardless of cleaner model type (two-way ANOVA F 1,23 =19.05, P <0.001; Fig. 3 ). There was no significant interaction between cleaner model type and confinement treatment on surgeonfish cortisol levels (two-way ANOVA F 1,23 =0.09, P =0.77; Fig. 3 ). In unconfined surgeonfish (that is, fish not exposed to an acute stress), which had access to moving models, cortisol level was not significantly correlated with the time fish had previously spent interacting with cleaner models (Spearman correlation: r s =0.37, n =7, P =0.40, Fig. 4a ). However, for confined surgeonfish (that is, fish exposed to an acute stress), which had access to moving models, cortisol levels decreased with increasing time previously spent interacting with models ( r s =−0.90, n =5, P =0.034, Fig. 4b ). 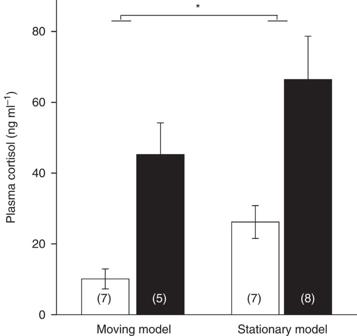Figure 3: The effect of receiving physical stimulation on cortisol levels of the surgeonfishC. striatus. Plasma cortisol levels of individual surgeonfishC. striatusthat had access to mechanically moving cleaner fish models or to stationary models. Within each group, surgeonfish were either exposed to a confinement stress test (confined group—black bars) or remained unconfined (unconfined group—white bars).P-values refer to significant differences between fish with access to physical stimulation or no access (* two-way ANOVA,P<0.05). Error bars represent ± 1 s.e.m. Sample sizes (number of individual surgeonfish) are given in parentheses. Figure 3: The effect of receiving physical stimulation on cortisol levels of the surgeonfish C. striatus . Plasma cortisol levels of individual surgeonfish C. striatus that had access to mechanically moving cleaner fish models or to stationary models. Within each group, surgeonfish were either exposed to a confinement stress test (confined group—black bars) or remained unconfined (unconfined group—white bars). P -values refer to significant differences between fish with access to physical stimulation or no access (* two-way ANOVA, P <0.05). Error bars represent ± 1 s.e.m. Sample sizes (number of individual surgeonfish) are given in parentheses. 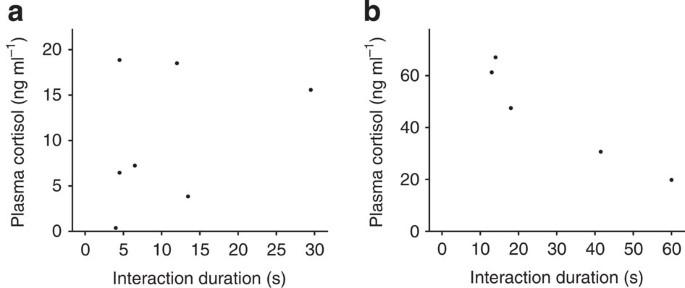Figure 4: The relationship between stress response and time previously spent receiving physical stimulation. The association between plasma cortisol levels and the time individual surgeonfish spent interacting (in seconds) with the moving mechanical cleaner wrasseL. dimidiatusmodel for: (a) surgeonfish that were not subjected to the confinement stress test (unconfined group) and, (b) surgeonfish that were confined before blood collection (confined group). Full size image Figure 4: The relationship between stress response and time previously spent receiving physical stimulation. The association between plasma cortisol levels and the time individual surgeonfish spent interacting (in seconds) with the moving mechanical cleaner wrasse L. dimidiatus model for: ( a ) surgeonfish that were not subjected to the confinement stress test (unconfined group) and, ( b ) surgeonfish that were confined before blood collection (confined group). Full size image Our study suggests that fish benefit, in the form of reduced stress, from physical contact alone. We found that physical stimulation by a cleanerfish model lowered basal cortisol levels in two ways: first, it reduced surgeonfish cortisol in controlled conditions regardless of exposure to a confinement stressor; and second, among individuals with higher levels of stress (confined group), variation in time previously spent receiving physical stimulation was significantly related with a decrease in the impact of an acute stressor ( Fig. 4b ). This revealed that physical contact, without any social factor, is enough to produce positive short-term physiological effects in fish, a phenomenon so far demonstrated only in humans [5] , [6] , [7] , [8] . Our results are thus in line with claims that the pathways for sensory information processing are more uniform among vertebrates than previously acknowledged [29] . Fish clients in the wild may combine this rewarding mechanism to a specific function: juvenile fish may learn to associate the seeking of cleaners and the receiving of physical contact to the relief of parasitism-derived tension or stress. However, parasitism would hardly be a reason for a rise of cortisol levels in the case of our experimental fish, as most parasites detach from their host during the process of capture and a re-infestation would be very unlikely under controlled conditions [30] . In the case of our experimental fish, similarly to other vertebrates in controlled housing conditions (farmed animals for example), stress might arise from social isolation and space limitations. In this case, physical contact by itself seems to function as a relevant stimulus for the reduction of stress. So far, the debate over somatic sensory systems in fish has mostly focussed on the neural processing and encoding of noxious stimuli (nociception) and pain perception. This has admittedly generated valuable information on the physiology of pain receptors and on fish individual's ability to change behaviour in response to noxious stimuli, with potential welfare implications for fish [31] , [32] . Our findings suggest that the somatic sensory system in fish is not only involved in nociception but that it is also involved in the processing of positive stimuli suggesting that future research should also focus on the role of physical contact on individuals' motivation to interact with others and on its potential health benefits. Our study may overturn the view of tactile stimulation by cleaner wrasses as a purely exploitative behaviour. Client parasite loads can vary tremendously among client species and from site to site [33] . As cleaners cheat more when few parasites are available on their clients [21] , some species with inherently low parasite loads may benefit little from interacting with cleaners. Our results suggest that cleaners can compensate clients for low cleaning quality by increasing tactile stimulation as an alternative mechanism to enhance client fitness in exchange for foraging opportunities (that is, client mucus). Accepting tactile stimulation may thus function as a successful coping strategy by clients to alleviate the effects of stress and enhance their health, which ultimately substantially contributes to the reciprocal nature of these interspecific interactions. Thus, our results propose a potential role of physical contact in the evolution and maintenance of mutualistic and social partnerships, and we suggest that future empirical research should explore further how it affects individual decision-making processes, and shapes animals' ability to respond to stressful experiences, as it is known to influence human behaviour [5] , [6] . Study species and housing conditions Experiments were conducted between June and July 2009 at the Lizard Island Research Station, Great Barrier Reef, Australia. All surgeonfish C. striatus were caught from the surrounding reefs and released at their site of capture after the experiments. These individuals are detritivores with small home ranges, are frequent clients to cleaning stations and readily adapt to captivity conditions [22] . A total of 32 surgeonfish were kept in groups of five to seven individuals in large, round holding tanks (1 m in diameter) with flow-through seawater for a minimum of 15 days before being transferred to individual experimental aquaria (64.5×41.3×39.7 cm) with flow-through seawater two days before the start of experiments. Several polyvinylchloride pipes (15 cm long and 16 cm diameter) served as shelter for the fish. The experiments were conducted sequentially in 16 aquaria. Experimental setup and behavioural observations To simulate tactile stimulation in the laboratory and to isolate the effect of physical contact from the multitude of other effects potentially resulting from interactions with cleaner fish, we developed an apparatus that allowed handmade, look-alike models of cleaner fish L. dimidiatus to move in a relatively realistic fashion ( Fig. 1 ; Supplementary Movie 1 ). Surgeonfish were categorized as small, medium or large, and equally distributed between treatments (mean±s.e., treatment fish standard length: 16.30±2.49 cm; control fish: 17.2±2.64 cm). Surgeonfish were then allocated to either a treatment group involving access to a moving cleaner model or a control group with access to a stationary cleaner model, using an alternate order between aquaria so that treatments would be equally distributed (experiments with individuals assigned to both groups were run simultaneously). On ten consecutive days, each fish was randomly exposed to one of the eight available models (four fish models were part of the four mechanical moving apparatus and four models were controls; see Fig. 1 ) for a total of 2 h (1 h in the morning and 1 h in the afternoon to include time of day effects). Trials were recorded with a video camera during the last day, while the experimenter left the site. We quantified the total cumulative number of events (frequency) and total duration of surgeonfish posing (which signals their willingness to interact [20] ), single-contact events and longer interactions during which the fish rubbed and was in continuous physical contact with the models. Of our initial sample size (32 fish), five fish were excluded from all analyses (behavioural and hormonal) as: one died before the conclusion of the exposures (confined, access to moving models), one remained inside its shelter during the entire experiment (unconfined, non-access to moving models), two never learned to approach and contact the moving models (confined, access to moving models) and one plasma sample was not in good condition (unconfined, access to moving models). Video recordings were analysed using the software package NOLDUS OBSERVER XT (Noldus Information Technology). Blood sampling procedure All blood collections took place on the morning of the 11th day. Before blood collection, half of the treated individuals and half of the control individuals were subject to a confinement stress test, which is a standardized method to measure acute stress responses in fish [27] . The confinement test entailed transferring each fish to a bucket (30 cm diameter) with a reduced amount of water (15 cm depth of water) for 30 min, followed by blood sampling. To collect blood, individuals from both groups were anesthetized by placing them in an aerated bucket with a solution of MS-222 in seawater (tricaine methanesulfonate, Sigma-Aldrich; dilution 1:10,000). After about 1 min, fish reached a deep stage of anesthesia [28] , [34] . A sample of 50 μl of blood was taken from the caudal vein. Fish were then placed in aerated water to recover from the anaesthesia for at least 5 min. The anaesthesia induction and blood sampling were performed within a maximum of 3 min, which is the latency for cortisol release into the systemic circulation in response to handling stress [35] . Hormonal analysis The free cortisol fraction was extracted from the plasma by adding diethylether as the steroid solvent. The samples were then centrifuged (5 min, 33.6 g , 4 °C) and frozen (10 min, −80 °C) to separate the ether fraction. The steroids were isolated by evaporating the ether. This process was repeated twice. Levels of free cortisol fraction were then determined by radioimmunoassay, using the commercial antibody 'Anti-rabbit, Cortisol-3' (ref: 20-CR50, Interchim (Fitzgerald), cross-reactivity: cortisol 100%, prednisolone 36%, 11-desoxycortisol 5.7%, corticosterone 3.3%, cortisone <0.7%) and the radioactive marker [1,2,6,7-3H] cortisol (ref: TRK407-250mCi, Amersham Biosciences). How to cite this article: Soares, M.C. et al . Tactile stimulation lowers stress in fish. Nat. Commun. 2:534 doi: 10.1038/ncomms1547 (2011).